Engineering protein thermostability using a generic activity-independent biophysical screen inside the cell Protein stability is often a limiting factor in the development of commercial proteins and biopharmaceuticals, as well as for biochemical and structural studies. Unfortunately, identifying stabilizing mutations is not trivial since most are neutral or deleterious. Here we describe a high-throughput colony-based stability screen, which is a direct and biophysical read-out of intrinsic protein stability in contrast to traditional indirect activity-based methods. By combining the method with a random mutagenesis procedure, we successfully identify thermostable variants from 10 diverse and challenging proteins, including several biotechnologically important proteins such as a single-chain antibody, a commercial enzyme and an FDA-approved protein drug. We also show that thermostabilization of a protein drug using our approach translates into dramatic improvements in long-term stability. As the method is generic and activity independent, it can easily be applied to a wide range of proteins. Methodologies to improve protein stability are of great importance for the biopharmaceutical industry. More efficient strategies of stabilizing proteins could potentially reduce efforts in protein manufacturing and formulation, as well as improve the safety of protein drugs. Biopharmaceuticals that have reached the clinic are generally highly thermostable [1] , [2] , [3] , [4] . In contrast, many protein drug candidates in development are suffering from poor stability [5] , [6] , which will affect efficacy and can lead to increased immunogenicity of the biopharmaceutical, inhibiting their advancement to the clinic. In several cases, these effects have been shown to arise from protein aggregation, often induced by exposure to ambient temperatures during protein handling or storage [7] , [8] . Similarly, biocatalysts used in a wide range of applications, such as in agriculture, paper, textile, the bio-energy industry or household care, are often highly stable at the conditions where they are applied. Unfortunately, in most cases the original enzyme is not directly suitable for the desired application because of the ‘hostile’ conditions at which the reactions are performed. For instance, thermal stability of biocatalysts is of major importance for industrial processes, since performing enzymatic reactions at high temperature has many advantages [9] , [10] . Therefore, during development, considerable engineering efforts are carried out to stabilize enzymes to increased temperatures [11] , [12] , [13] , [14] . Protein stability is also of great importance in basic research, as stable proteins are more amenable to biochemical and structural studies. Thermal stability has, for instance, been shown to increase the likelihood of crystallization of both soluble and membrane proteins. This concept is now one of the most promising avenues on the path to obtain crystal structures of challenging proteins, such as G protein coupled receptors [15] , [16] and protein kinases [17] . In addition, in the field of directed evolution and protein engineering improved thermostability of the target is usually desirable since it correlates with the mutational robustness of the target: destabilizing mutations, that are necessary for a new activity, are more easily tolerated [18] . For all the applications mentioned above, understanding and improving protein stability through directed evolution is a key strategy. Current approaches rely on an indirect read-out of protein stability, typically a functional assay after a stability challenge. For enzymes, for example, a heating step is typically performed, followed by a read-out of residual activity in multi-well plates [10] . For proteins able to bind with relatively strong affinity to a target, such as antibodies, a denaturation step can be followed by a read-out on residual binding [19] , [20] . There are many successful examples in the literature of this type of approaches; however, their customized nature limits the number of targets that can be evolved in parallel. Directed evolution is therefore usually restricted to specialized research teams working on a small number of proteins. Moreover, as the number of sequenced genomes is expanding rapidly, many research fields have streamlined their research structure to be able to study as many proteins as possible in a high-throughput manner, for example, protein production, purification and structural biology [21] , [22] . The study and improvement of protein stability through directed evolution approaches has not made that transition yet, as there are no generic, streamlined techniques for this purpose. There have been attempts to develop generic (thermo)stability screens that are independent of protein function, that allow the study of many different targets in parallel and have enough throughput to screen libraries of significant size: these include Proside [23] , THR [24] and the tripartite fusion system [25] . However, these methods are handicapped by indirect read-outs of thermostability, which increases the risk for false positives or negatives, and their general applicability is yet to be demonstrated. Here we develop a broadly applicable, high-throughput and activity-independent method to study and increase protein thermostability. The method is an extension and modification of our previously published colony filtration (CoFi) blot method [26] . It circumvents most of the problems linked to current stability selection methods while expanding its applicability to virtually any protein target that can be expressed recombinantly in a colony-forming microorganism. We show that the method can be used to accurately determine the intrinsic protein-melting temperatures in cells and is an effective screening technology to identify more stable variants of a target protein in directed evolution experiments. Importantly, we present a clear, streamlined process that allows studying and evolving several targets in parallel with no optimizations required. The wide applicability and potential of this method is demonstrated on a broad range of targets representing protein drugs, biotechnology tools, enzymes and challenging structural biology targets. Thermal stress leads to protein aggregation in vivo Thermal stress of a purified protein above a certain critical temperature usually leads to irreversible protein unfolding, followed by rapid aggregation [27] . We hypothesized that a similar scenario might be in effect for recombinant proteins overexpressed in Escherichia coli , and that this could be utilized to select more stable proteins. When cells are subjected to increased temperatures, the proteins might unfold and aggregate in a similar way as purified proteins. We selected a set of nine proteins with a midpoint of unfolding (melting temperature; T m ) of the purified protein ranging from 40 °C to 68 °C, which were cloned into expression plasmids, transformed into E. coli and plated. The colonies were then transferred to a filter membrane that previously has been shown to let soluble proteins pass through while retaining aggregates [26] . After expression, the colonies were incubated at a wide range of temperatures after which they were subjected to concurrent lysis and CoFi [26] ( Fig. 1a,b ). In this step, the filter membrane retains aggregates, while soluble proteins diffuse from the lysed colonies onto a nitrocellulose membrane. The protein is then detected using affinity reagents against the target itself or against a detection tag fused to the target. A high signal indicates the presence of soluble protein, while signal loss accounts for protein aggregation in the cell. For all proteins tested, there was a good correlation between signal loss and the T m determined by differential scanning fluorimetry (DSF) that measures the unfolding of the purified proteins ( Fig. 1c ) [28] . This correlation strongly indicates that it is the unfolding and subsequent aggregation of the protein inside the cell that we are measuring. We therefore consider our screen to be a biophysical screen, analogous to differential static light scattering [29] , setting it apart from previously published thermostability screens used for directed evolution of stability. Interestingly, the midpoint of the cellular aggregation curve (named here T cagg ) was generally a few degrees lower than the T m obtained by DSF ( ∼ 5 °C lower on average). This difference might reflect the influence of the macromolecular crowding of the cell on protein in vivo thermal stability. The wide temperature range accessible by the method covers the T m of most mesophilic proteins, making the method widely applicable. 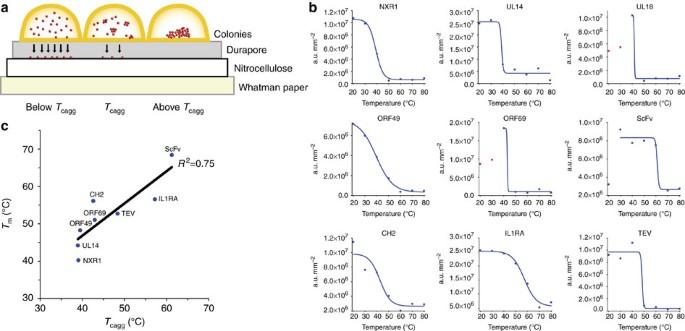Figure 1: Determination of the temperature of cellular aggregation (Tcagg) of diverse proteins by Hot-CoFi. (a) Schematic representation of the Hot-CoFi method. Below theTcagg, proteins are soluble and are able to diffuse through the Durapore membrane and bind the nitrocellulose membrane. As temperature is increased, more proteins aggregate, leading to a reduction of diffusion towards the nitrocellulose. (b) Cellular aggregation curves obtained using Hot-CoFi. Signals obtained represent chemoluminescence signal in arbitrary units (a.u.) from the whole colony, and standardized in mm2to account for colony size. Blue dots represent the signals obtained and used for the fitting of sigmoidal curves. Red dots were excluded from the curve fitting; for UL18 and ORF69, they correspond to very intense signals that burned all the substrate on the membrane, leading to an apparent weaker signal. (c) Comparison of melting temperatures (Tm) obtained by DSF againstTcaggobtained by Hot-CoFi. UL18 is not included as it was not possible to determine itsTm. (n=1). Figure 1: Determination of the temperature of cellular aggregation ( T cagg ) of diverse proteins by Hot-CoFi. ( a ) Schematic representation of the Hot-CoFi method. Below the T cagg , proteins are soluble and are able to diffuse through the Durapore membrane and bind the nitrocellulose membrane. As temperature is increased, more proteins aggregate, leading to a reduction of diffusion towards the nitrocellulose. ( b ) Cellular aggregation curves obtained using Hot-CoFi. Signals obtained represent chemoluminescence signal in arbitrary units (a.u.) from the whole colony, and standardized in mm 2 to account for colony size. Blue dots represent the signals obtained and used for the fitting of sigmoidal curves. Red dots were excluded from the curve fitting; for UL18 and ORF69, they correspond to very intense signals that burned all the substrate on the membrane, leading to an apparent weaker signal. ( c ) Comparison of melting temperatures ( T m ) obtained by DSF against T cagg obtained by Hot-CoFi. UL18 is not included as it was not possible to determine its T m . ( n =1). Full size image Evolution of protein thermostability The efficiency of our method (hereafter referred to as Hot-CoFi) to assess protein-melting temperatures in cells encouraged us to implement it as a screen for improvement of thermostability using directed evolution approaches. A diverse set of proteins was chosen for stabilization, representing several main applications where protein stability is crucial. For biotechnology and biopharmaceutical applications, a single-chain Fv (scFv) antibody (against Grb2-SH2 domain, based on Genentech’s 4D5 scaffold), interleukin-1 receptor antagonist (IL1RA, Anakinra, developed by Amgen for rheumatoid arthritis treatment) and immunoglobulin VH and CH2 domains (currently developed as new scaffolds for binder generation [30] , [31] ) were chosen. For structural biology, NXR1 (the NUDIX hydrolase domain of human NUDT18) and numerous viral proteins (commonly characterized by loosely packed cores and unstructured regions) [32] were selected. Finally, for biocatalyst stabilization applications, a highly specific cysteine protease was used as a model protein, the tobacco etch virus (TEV) protease ( Table 1 ). Table 1 Description of targets stabilized. Full size table For all targets, random mutagenesis libraries were generated using error-prone PCR in combination with library cloning using megaprimer PCR of whole plasmid (MEGAWHOP) [33] . The libraries were screened using Hot-CoFi at a temperature of ∼ 5 °C–10 °C above T m for the wild-type (WT) protein ( Fig. 2a ). Colonies with a chemiluminescence signal intensity three times stronger than that of the background colonies were judged to be positive ( Supplementary Fig. S1A ). The variation in intensity between the negative colonies are typically very small, usually with a s.d. that is 10% of the average intensity ( Supplementary Fig. S1B ). Positive clones were further verified by re-streaking the picked colonies and re-screening using the Hot-CoFi blot, with WT as a control. Clones that were positive in the second screen were produced in large scale and purified by immobilized metal ion affinity chromatography (IMAC) and size exclusion chromatography (SEC). To determine the T m of the purified proteins, DSF [28] was performed and to determine the midpoint of aggregation ( T agg ) differential static light scattering was used [29] . 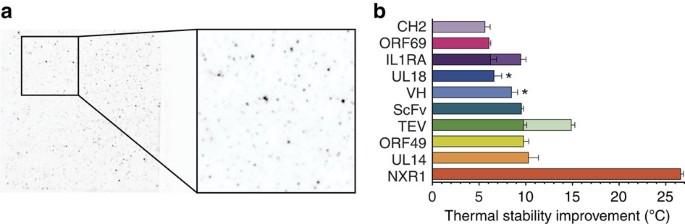Figure 2: Evolving protein thermal stability by random mutagenesis and Hot-CoFi screening. (a) Typical result obtained from screening a random mutagenesis library by Hot-CoFi. Dots with high intensity represent colonies expressing stable variants of the target protein. (b) Thermal stability improvement obtained for the best mutant of each target (and corresponding s.d.). For all targets, DSF values are shown, except for UL18(*) and VH domain(*) for which differential static light scattering had to be used because of poor behaviour in DSF. Error bars, s.d. (n=3). Figure 2: Evolving protein thermal stability by random mutagenesis and Hot-CoFi screening. ( a ) Typical result obtained from screening a random mutagenesis library by Hot-CoFi. Dots with high intensity represent colonies expressing stable variants of the target protein. ( b ) Thermal stability improvement obtained for the best mutant of each target (and corresponding s.d.). For all targets, DSF values are shown, except for UL18(*) and VH domain(*) for which differential static light scattering had to be used because of poor behaviour in DSF. Error bars, s.d. ( n =3). Full size image Virtually all of the clones selected after the confirmation screen were also more thermostable after purification (95% of positives that were purified and for which a T m or T agg was obtained), and the range of improvement in thermal stability after just one round of mutagenesis ranged from 5.6 °C to 26.6 °C with a median of 9 °C for the best mutants ( Fig. 2b . See Supplementary Table S1 for a complete list of positive mutants obtained and their corresponding stability, and Supplementary Fig. S2 for in vitro thermal shift curves of WT and best mutants). For many of the targets, we also further characterized the biophysical and biochemical properties of the mutants and compared them with WT. Evolution of protein thermostability for structural biology Initial thermostabilization studies were performed on NXR1 (PDB ID 3GG6). This human protein domain represents a typical structural biology target for which the structure was previously solved at a resolution of 2.1 Å using the multi-construct approach. After screening ∼ 5,000 clones using Hot-CoFi, three stabilized mutant proteins were obtained. The largest improvements of T m was 26.6 °C for mutant NXR1-1, arising from two mutations. In this case, one mutation actually targets the active site, and is therefore likely to abolish activity. NXR1 WT and mutants were subjected to crystallization trials. Minimal crystallization efforts yielded a crystal diffracting to 1.5 Å for the most stable mutant (NXR1-1), without requiring ligand stabilization or optimization of crystallization conditions ( Supplementary Fig. S3 , Supplementary Table S2 ). This is in line with previous reports suggesting that thermal stabilization leads to increased likelihood of crystallization and better diffraction data [15] , [16] , [34] . Stabilizing biotechnology tool proteins and protein drugs scFv antibody fragments are important tools in modern biotechnology. They are, for example, used in library-based generation of renewable binders [35] , which can be further developed into intact antibodies and protein drugs. ScFv also have direct potentials as protein drugs owing to improved pharmacokinetics for tissue penetration as compared with IgGs [36] . However, the stability of scFvs can vary widely, which often compromises their usefulness in medical applications and as biotechnology tools [37] . Hot-CoFi screening of random mutagenesis libraries of anti-Grb2 scFv, based on 4D5 scaffold (anti-Her2 IgG, Herceptin), produced several stabilized mutants, the best of which has a T m that is 9.5 °C higher than WT. The analysis of the mutations ( Supplementary Fig. S4 ) suggests CDR-H3 as a hotspot for stabilizing mutations. Indeed, five out of eight stable variants isolated by Hot-CoFi contain mutations in this loop, highlighting its critical role for scFv stability. There also seems to be a hotspot for stabilizing mutations in the first 10 residues of the sequence, suggesting the amino terminus as a potential target to further improve stability using more site-directed libraries. To confirm that the stabilized mutants retained the affinity of the WT, the affinity against the Grb2-SH2 domain was characterized by surface plasmon resonance (SPR; Supplementary Fig. S5 ). Most mutants retained a binding affinity similar to WT. However, the most stable variant (scFv-1), containing a single mutation (W225G) in CDR-H3, lost considerable binding affinity from an original ∼ 50 pM for WT to >43 nM. The reduction in binding affinity of this mutant might be due to the adoption of a new conformation by CDR-H3 that is not favourable for Grb2 binding. Protein drug stability is critical for their therapeutic application, as low stability hampers their efficacy and safety. IL1RA was chosen as a test example for the stabilization of a protein drug as it is biopharmaceutically characterized by an aggregation propensity linked to poor thermal stability [38] , [39] . Therefore, extensive efforts have been made to improve the stability of IL1RA by reformulation [40] in conjunction with studies of longer-term storage and thermal stability [38] , [39] , [41] . A first cycle of random mutants of IL1RA were produced and screened for improved stability. Four mutant proteins were isolated, all having a stability improvement of ∼ 6 °C over WT. All positive mutants were combined for a second cycle with additional random mutagenesis followed by stability screening. Five new mutants were obtained with improved stabilities of up to 9.5 °C over WT. These variants contain mutations combined from the four different first cycle-stabilized clones ( Supplementary Table S1 ). The most stable mutant, IL1RA-8 (round 2), combines one mutation from IL1RA-1 (A12T) and two mutations from IL1RA-2 (H54N, F148L). To assess whether the mutations affect binding against type I IL1 receptor (IL1R), WT, IL1RA-2 (round 1) and IL1RA-8 (round 2) were further characterized by SPR. Both mutants have a similar K D against IL1R compared with WT ( Supplementary Fig. S6 ), with a final equilibrium dissociation constant, K D of 550 pM for IL1RA-8 (290 pM for WT). Subsequently, we mapped the mutated residues of IL1RA-8 in the IL1RA-IL1R complex structure ( Fig. 3a ). The mutations cluster in the opening of IL1RA beta-barrel, suggesting that this area is favourable for stabilization. As can be seen in the structure, they are located far from the interaction site with IL1R domains one and two, but in proximity of the interaction site with domain three. A12 and F148 do not participate in this interaction, while H54 interacts with IL1R’s T297 through main chain to main chain interactions [42] . Interestingly, in the IL1RA apo structure, H54 has no side-chain density and is part of a partially disordered loop comprising residues 51–54 (ref. 43 ). This particular loop changes conformation and is stabilized on receptor binding [42] . H54N might thus contribute to the marginal reduction of binding. Other stabilized variants contain mutation P50H, a mutation that confirms the importance of this loop for stability. New mutations in this area might allow the selection of further stabilized variants with retention or improvement of affinity. 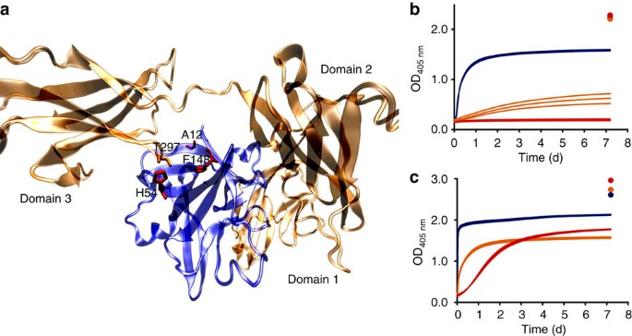Figure 3: Characterization of IL1RA and its variants. (a) Structure of IL1RA (blue) complexed with IL1R (orange), from PDB ID 1IRA. IL1RA residues A12, H54 and F148 are highlighted in red; IL1R residue T297 is highlighted in orange. (b,c) Stability of IL1RA and mutants. Aggregation is measured at OD405 nm, at a protein concentration of 50 mg ml−1, and at a temperature of 30 °C (b) or 40 °C (c). WT is in blue, IL1RA-2 in orange and IL1RA-8 in red. After 7 days, the samples were heated at 80 °C for 30 min to obtain the maximum aggregation signal (filled circles) (n=3). Figure 3: Characterization of IL1RA and its variants. ( a ) Structure of IL1RA (blue) complexed with IL1R (orange), from PDB ID 1IRA. IL1RA residues A12, H54 and F148 are highlighted in red; IL1R residue T297 is highlighted in orange. ( b , c ) Stability of IL1RA and mutants. Aggregation is measured at OD 405 nm , at a protein concentration of 50 mg ml −1 , and at a temperature of 30 °C ( b ) or 40 °C ( c ). WT is in blue, IL1RA-2 in orange and IL1RA-8 in red. After 7 days, the samples were heated at 80 °C for 30 min to obtain the maximum aggregation signal (filled circles) ( n =3). Full size image In light of these results and the potential therapeutic application of these variants, accelerated stability studies were performed using buffer conditions and concentrations similar to the formulation of the clinical version of IL1RA, Anakinra [39] . The best first- and second-cycle mutants (IL1RA-2 and IL1RA-8, respectively) were compared with WT protein in a thermal challenge in CSE buffer, at a concentration of 50 mg ml −1 over 1 week at 30 °C, measuring aggregation spectrophotometrically at 405 nm ( Fig. 3b ). In these conditions, the WT protein starts to aggregate after 2 h, IL1RA-2 after ∼ 10 h, while IL1RA-8 shows no sign of aggregation even after 7 days. Equivalent long-term stability experiments were performed at 40 °C ( Fig. 3c ). WT started aggregating after 25 min and had aggregated completely in 1 h. IL1RA-2 started aggregating at a similar time point (33 min), but aggregated at a slower rate, leading to a plateau only after 2 days. IL1RA-8 started to aggregate only after 5–10 h, and reached a plateau after 4 days. Stabilization of enzymes To study the usefulness of the Hot-CoFi method for stabilization of biotechnologically important enzymes, the TEV protease was chosen as a test case. For this target, 17 positive clones were obtained, with stability improvements of up to 9.8 °C. Activity experiments were carried out at room temperature (RT) to compare the performance of these stabilized variants against WT. Most mutant proteins maintained identical activity to the WT ( Supplementary Fig. S7 ). Five active and diverse variants (mutants TEV-1, TEV-6, TEV-8, TEV-14 and TEV-17) were selected for a new cycle of random mutagenesis library creation and screening. Twenty-two variants were obtained with up to 14.9 °C improvement in stability over WT. Eight of these were fully active ( Supplementary Fig. S8 ). When heat challenged at 60 °C for 20 min before performing activity assays, the WT protein was inactive, while the most stable first- and second-cycle mutants were partially and fully active, respectively ( Supplementary Fig. S9 ). The sequences of all the stabilized second-cycle mutants were analysed, and the frequency of each mutation was calculated. The most conserved mutations were highlighted on TEV protease structure in Fig. 4 . E119G is the most conserved mutation (frequency of 94%), followed by L251S (78%), N25S (44%) and S170A (28%). The most stable variant, TEV-35 (round 2), combines the three most frequent mutations: one from TEV-6 (E1119G) and two from TEV-8 (N25S, L251S). In addition, it contains one mutation from TEV-17 (Q87L) plus one new mutation (L7S). Interestingly, the three most stable active variants, TEV-35, TEV-20 and TEV-26, contain mutations Q87L, T84A and F53L, respectively, all located in the same small hydrophobic core, suggesting that this area might be amenable for further stabilization without compromising TEV protease activity. 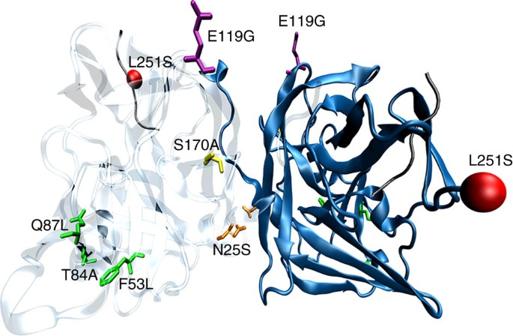Figure 4: TEV structure sheds light into the stabilization effect of mutations. TEV structure (PDB ID 1LVM) is shown in blue (chain A is opaque and chain B is transparent). E119G is highlighted in purple, L251S as a red sphere at the C terminus (as the residue is missing in the structure), N25S is in orange and S170A is in yellow. Q87L, T84A and F53L are in green. TEV digestion product (which indicates the active site) is shown in grey. Figure 4: TEV structure sheds light into the stabilization effect of mutations. TEV structure (PDB ID 1LVM) is shown in blue (chain A is opaque and chain B is transparent). E119G is highlighted in purple, L251S as a red sphere at the C terminus (as the residue is missing in the structure), N25S is in orange and S170A is in yellow. Q87L, T84A and F53L are in green. TEV digestion product (which indicates the active site) is shown in grey. Full size image Although our screen does not report on the enzymatic activity of the target, we found several clones for the TEV protease that retained a similar activity as compared with WT, indicating that our method could be a potential route to obtain heat-resistant enzymes without compromising activity. By pre-screening and enriching libraries with thermostable variants before performing functional assays, the screening power can be increased while reducing costs. We describe a new method to study thermal stability of overexpressed proteins in cells, and its use for the screening of stabilized protein variants using a directed evolution approach. Our method is rapid, robust and efficient in detecting stabilized proteins. The method is effective over a wide range of screening temperatures and is generic as it is potentially applicable to most soluble proteins expressed in a colony-forming microorganism. Our method has several advantages to existing activity-independent thermostability screens available, that is, Proside [23] , THR [24] and the tripartite fusion system [25] , thanks to its direct biophysical stability read-out and broad applicability. Proside [23] is a phage-based method that relies on an indirect read-out of protein folding through protease resistance and phage infectivity rather than thermostability. Moreover, the need to display the protein on the bacteriophage’s surface considerably limits the number of targets amenable to the technique. THR [24] is based on the expression of a thermostable variant of kanamycin nucleotidyl transferase fused to the target gene in Thermus thermophilus . However, the host used is not a validated recombinant protein expression system, and the screening temperature window is narrow (60–75 °C). The tripartite fusion system [25] is based on a split β-lactamase containing the target gene inserted between the two fragments and expressed in E. coli . It is not a thermostability screen per se but rather a ‘foldability’ and protease resistance screen without temperature challenge. Further, it requires the correct insertion of the target gene in between the two fragments of the reporter. Moreover, none of these methods have become the standard way of generating more stable variants of a target protein. We have demonstrated the broad applicability of our method by generating more thermostable variants of 10 diverse proteins, as well as exemplified potential applications. The simplicity of the method allows it to be used by any laboratory, requiring only standard laboratory equipment. Many targets can be evolved in parallel, with a throughput of up to ∼ 100,000 clones per experiment (that is, screening five to six plates with a density of 15,000–20,000 colonies per plate). This represents a significant advantage of our method over existing alternatives, as the study and evolution of many targets in parallel dramatically increases the throughput. Furthermore the simplicity of the process allows its widespread use by laboratories not specialized in directed evolution. The fact that we can confirm the improved stability of 95% of all characterized clones at the level of purified proteins highlights the excellent stringency and robustness of the method. From previous work in the literature, typical stabilizations obtained, in the first round of selection, is in the range of 2–5 °C (refs 11 , 12 , 13 , 14 ) and the stabilization seen in our experiments is two to three times better than these (median stabilization is 9 °C). The excellent performance of Hot-CoFi in identifying stabilizing mutants is likely to arise from the direct read-out of thermostability, as well as a relatively large screening capacity. We believe that our stability screen is the preferred option when no functional assays are available for a potential target protein. All of the structural biology targets studied here have no activity assay available, and were successfully stabilized with Hot-CoFi. Moreover, our screen allowed the stabilization of several viral proteins, including the viral capsid protein UL18, suggesting Hot-CoFi as a new tool for recombinant vaccine development. The characterization of IL1RA, TEV and scFv highlights the great potential of Hot-CoFi to improve the stability and biophysical properties of biopharmaceuticals and biotechnological proteins. Resistance to aggregation either by heat stress or long-term storage at room temperature would be of great benefit for both biotech and biopharma industries, as it increases the possible industrial applications of biologics for the former, and the safety and formulation options for the latter. We believe our method has great potential applicability in both industries for such purposes. In addition, we believe that our method can be of great value in the field of directed evolution, as it could be used to generate stable parents/scaffolds with increased mutational robustness before protein engineering efforts are carried out. Finally, for many of the targets (NXR1, IL1RA, scFv and TEV), Hot-CoFi automatically identified hotspots in the protein where stabilizing mutations are clustered. This seems to indicate that the data generated with this method will also shed light on fundamental aspects of protein stability. Cloning of the target genes UL14 , UL18 , ORF49 and ORF69 genes were kindly provided by Dr Jurgen Haas (University of Edinburgh), anti-Grb2 scFv gene was kindly provided by Dr Sachdev S. Sidhu (University of Toronto) and a solubility-improved variant of TEV protease [44] was provided by Dr Helena Berglund (Karolinska Institute). IL1RA (isoform 2), 4D5 VH domain, CH2 domain and TEV-SUMO-TEV were synthesized (Genscript), while NXR1 was cloned from the human mammalian gene collection. All the genes studied were subcloned by ligation-independent cloning (LIC) [45] , with the exception of TEV protease, which was already provided in a suitable vector. For LIC cloning, the destination vector was pNIC-CH3, a pET-based expression vector containing a carboxy-terminal His 6 tag (TEV protease was in pTH-24). The genes were amplified by PCR using gene-specific primers that contained universal LIC forward (5′-AGAGGAGATAATTA-3′) and LIC reverse (5′-AATGGTGGTGATGATGGTGCGC-3′) overhangs. Treatment of the insert and the linearized vector with T4 DNA polymerase, in the presence of only dCTP or dGTP, respectively, generates 15-nucleotide-long overhangs by the polymerase’s 3′-exonuclease activity. T4 polymerase-treated insert and vector were annealed, and used to transform a bacterial cloning strain. The presence of a negative selection marker gene, SacB (coding for B. subtilis levansucrase, conferring sensitivity to sucrose), in pNIC-CH3 vector between two Bfu AI sites (excised after vector linearization) allows the selection of the vector containing the desired gene on LB agar plates in the presence of 50 μg ml −1 kanamycin and 5% sucrose. Temperature of cellular aggregation The T cagg was determined following a modified protocol based on the CoFi blot [26] , [46] . Rosetta2 cells (Novagen) were transformed with the expression plasmids, harbouring the gene of interest fused with a C-terminal His 6 -tag, and the cells were plated. Individual colonies were picked and grown overnight at 37 °C in terrific broth supplemented with antibiotics (50 μg ml −1 kanamycin or ampicillin, according to the vector, and 34 μg ml −1 chloramphenicol). Two microlitre aliquots of culture were plated in as many LB agar plates+antibiotics as temperatures to screen and incubated at 37 °C until a lawn was visible. Colonies were transferred to a Durapore 0.45 μm filter membrane (Millipore) and placed on LB agar plates (colonies facing up) supplemented with antibiotics and 0.2 mM isopropyl β- D -1-thiogalactopyranoside (IPTG), except for the single-chain antibody, VH domain and IL1RA, for which 1, 25 and 30 μM IPTG were used, respectively. Induction was performed overnight at RT for protein expression. After protein production, the induction plates were incubated at temperatures ranging from 20 to 80 °C, with temperature intervals of 10 °C, for 30 min. In the meantime, a lysis sandwich was prepared, composed of a Whatman paper, soaked in CoFi lysis buffer (20 mM Tris, pH 8.0, 100 mM NaCl, 0.2 mg ml −1 lysozyme, 11.2 U ml −1 Benzonase endonuclease (Merck) and 1:1,000 dilution of Protease Inhibitor Cocktail Set III, EDTA-Free (Merck)), and a nitrocellulose membrane (Millipore). The lysis sandwich was incubated 10 min at the screening temperature. The Durapore membrane was then transferred on top of the lysis sandwich, with the colonies facing up, and incubated at the screening temperature for another 30 min. Cells lysis was further improved by three freeze-thaw cycles at −80 °C and RT, respectively (30 min each). The Durapore membrane and the Whatman paper were discarded, and the nitrocellulose membrane was incubated in blocking buffer (TBS-T buffer (20 mM Tris, pH 7.5, 500 mM NaCl, 0.05% (vol/vol) Tween 20) and 1% BSA) for 1 h at RT. After blocking, the nitrocellulose membrane was washed three times in TBS-T, 10 min at RT, with shaking at 70 r.p.m. It was then incubated in TBS-T containing a 1:5,000 dilution of HisProbe-HRP (Thermo Scientific), for 1 h at RT, with shaking at 30 r.p.m. Three washing steps were followed and performed as mentioned above. The nitrocellulose membrane was developed using Super Signal West Dura chemiluminescence kit (Thermo Scientific), using a charge-coupled device camera (Fujifilm LAS-4000). Signal intensities were measured using Multi-Gauge software (Fujifilm) over the area corresponding the colonies and normalized by area (unit: arbitrary intensity units per mm 2 ). Library generation Error-prone PCR was performed using Genemorph II Mutagenesis Kit (Stratagene), using the cloned genes as template, according to the manufacturer’s protocol. An average of 50 ng of insert template was used, in a 30-cycle PCR reaction with phosphorylated primers, leading to an average of approximately two to three amino-acid mutations per gene in the final plasmid library. The error-prone PCR product was gel purified (Qiagen Gel purification Kit). The plasmid library was created by MEGAWHOP reaction [33] , using an optimized protocol described here. Typically, 1–10 ng of plasmid containing the WT gene was used as template, and amplified using ∼ 1 ng of insert per bp of insert length of purified epPCR insert as megaprimer (for example, 500 ng for a 500-bp insert) in a PCR reaction with KOD Xtreme polymerase (Merck). The buffer composition was the standard recommended by the manufacturer, with the addition of 1 mM NAD+ and 40 U of Taq DNA ligase, and using 0.5 U of KOD Xtreme polymerase. The PCR conditions were as follows: 94 °C for 2 min, (98 °C for 10 s, 65 °C 30 s, 68 °C for 6 min) for 30 cycles, 4 °C on hold. After PCR, 20 U of Dpn I (NEB) was added to the PCR reaction, and incubated for 3 h at 37 °C. DH10B cells were electroporated with the Dpn I-treated MEGAWHOP product yielding libraries of ∼ 10 5 unique members. Library screening Rosetta2 cells were transformed with the mutagenesis libraries, and plated on 24.5 cm diameter square LB agar plates supplemented with 50 μg ml −1 kanamycin (ampicillin, for TEV protease) and 34 μg ml −1 chloramphenicol. These are considered master plates. They were screened using the same protocol as described for T cagg determination, but at a single temperature, typically 5–10 °C above the purified protein’s T m or T agg for 30 min. VH domain was an exception, as it was screened at 80 °C (16 °C above T agg ), the induction plate being incubated for 1.5 h at that temperature. Positives colonies were selected according to signal intensity (three times more intense than ‘background colonies’), and picked from the master plate. To avoid cross-contaminations or false positives, each picked colony was re-streaked onto Agar plates and four new colonies picked from the re-streak. They were verified by regrowing them as 2 μl bacterial lawns, and repeating the same screening procedure, and including the WT clone as a control. Positive mutants, confirmed from the verification step, were produced in large scale for biophysical characterization. Protein production and purification Selected positive clones were produced in large-scale cultures using 0.75 or 1.5 l of terrific broth (TB)+antibiotics, and incubated at 37 °C using a LEX bioreactor system (Harbinger Biotechnology & Engineering). When OD 600 nm reached 2, the culture was cooled to 18 °C for 30 min, protein production was induced with 0.5 mM IPTG (except for IL1RA, VH domain and ScFv, induced with 25, 30 and 1 μM IPTG, respectively) and incubated overnight at 18 °C. For long-term stability experiments performed for IL1RA at high concentration, protein production was performed in a larger scale. For WT, 12 l of TB+antibiotics were used, while 6 l were used for each mutant. Cultures were harvested by centrifugation at 4,000 g , 25 min at 4 °C. The pellets were weighed and solubilized in 1.5 volumes per weight of pellet lysis buffer (100 mM HEPES, pH 8.0, 500 mM NaCl, 10 mM imidazole, 10% glycerol). Cells were lysed by performing one cycle of freeze thawing at −80 °C and RT, followed by sonication. The lysed cells were centrifuged at 46,000 g , for 25 min at 4 °C, the supernatant was collected and filtered through a 1.2-μm filter syringe. The filtrate was then purified by IMAC, followed by SEC. The IMAC column (Ni-NTA Agarose, Qiagen) was washed with 20 column volumes of IMAC wash-1 buffer (20 mM HEPES, pH 7.5, 500 mM NaCl, 10 mM imidazole, 10% glycerol), followed by 20 volumes of IMAC wash-2 buffer (20 mM HEPES, pH 7.5, 500 mM NaCl, 25 mM imidazole, 10% glycerol). The desired protein was eluted with five column volumes of IMAC elution buffer (20 mM HEPES, pH 7.5, 500 mM NaCl, 500 mM imidazole, 10% glycerol). The IMAC eluate was loaded onto a Superdex-75 or Superdex-200 SEC column (GE Healthcare) according to protein size, for further purification, and eluted in SEC buffer (20 mM HEPES, pH 7.5, 300 mM NaCl, 10% glycerol). Tris-(2-carboxyethyl)phosphine was added to all the purification buffers to a final concentration of 0.5 mM. For the VH domain, IMAC purification was performed as described, but further purified using a 1 ml HiTrap rProtein A FF column (GE Healthcare). To do so, the protein A column was equilibrated with 10 ml of SEC buffer and the IMAC eluate was loaded. The column was washed with 10 ml of SEC buffer. The protein was eluted with 0.1 M glycine, pH3 and neutralized by 1:5 v:v of neutralization buffer (1 M Tris, pH8, 1.5 M NaCl, 10% glycerol). For long-term stability experiments performed for IL1RA, purification followed the standard IMAC and SEC purification procedures, but for SEC, the buffer was changed to CSE buffer (10 mM sodium citrate, 140 mM NaCl, 0.5 mM EDTA, pH 6.5). Biophysical characterization The denaturation temperature of the purified protein variants was determined by DSF, except for UL18 and VH domain for which differential static light-scattering was used instead, according to published methods [29] , [34] . To perform DSF, 5 μg of the proteins were diluted into a 25-μl SEC buffer solution containing 5 × SYPRO Orange fluorescent dye (Bio-Rad). Proteins were tested in triplicates, the fluorescence was monitored using a 96-well Real-Time PCR detection system (iCycler iQ, from Bio-Rad), from 25 to 95 °C, with a gradual temperature increase of 1 °C every 10 s. For differential static light-scattering experiments, 5 μg of protein was diluted into 50 μl of SEC buffer (for VH domain, 1 mg ml −1 of protein was used instead to obtain aggregation curves) and dispensed in triplicates in 384-well optical bottom plates with black upper structure (Nunc). The samples were sealed with 50 μl of mineral oil (Sigma-Aldrich) and centrifuged at 15 °C, 3 min at 3,200 g . Static light scattering was monitored using a differential static light scattering detection system (StarGazer from Harbinger Biotechnology & Engineering) in a temperature range of 25–80 °C, with a gradual increase in temperature of 1 °C min −1 . The T m and T agg were determined using the Boltzmann equation, by the instrument’s software. Crystallization and structural determination NXR1 WT and mutants were used in crystallization trials at a concentration of 10 mg ml −1 by sitting-drop vapour diffusion on a three-well Intelli-plate96 (Art Robbins Instruments) using the JCSG+ Suite screen (Qiagen) and incubated at room temperature. Mutants 3 and 5 gave crystals in 0.1 M tri-sodium citrate, pH 5 and 3.2 M ammonium sulphate. Mutant 5 crystals were mounted and frozen. Diffraction data were collected at the National Synchrotron Radiation Research Center (Taiwan), using beamline 13B1, a wavelength of 1.0 Å, and a temperature of 100K. The structure was solved and refined using CCP4 suite [47] and Phenix [48] by molecular replacement using PDB 3GG6 as a template. Ramachandran statistics obtained are the following: Ramachandran favoured 99%, outliers 0%, clashscore 11.07. Structure data collection and refinement statistics are presented in Supplementary Table S2 . Surface plasmon resonance IL1RA and anti-Grb2 ScFv were characterized by SPR against their targets IL1 receptor (R&D Systems) and Grb2-SH2 domain, respectively. The Biacore T-3000 (GE Healthcare) and CM5 amine-coupling chips (GE Healthcare) were used following the manufacturer’s recommendations. For IL1RA, WT and mutants were immobilized at ∼ 400 response units. IL1 type I receptor was injected in SPR buffer (10 mM HEPES pH 7.4, 150 mM NaCl, 3.4 mM EDTA, 0.005% surfactant P-20) at a flow of 30 μl min −1 for 6 min, followed by a dissociation period of 1 h. Remaining bound protein was dissociated with 15 μl of 20 mM HCl. For anti-Grb2 ScFv, Grb2-SH2 domain was immobilized at ∼ 80 response units. ScFv WT and mutants were injected in SPR buffer at a flow of 30 μl min −1 for 2 min, followed by a dissociation period of 10 min. Remaining bound protein was dissociated with 15 μl of 20 mM HCl. Long-term stability study for IL1RA Long-term stability studies were performed for IL1RA WT and mutants in CSE buffer, at a protein concentration of 50 mg ml −1 (ref. 39 ). For experiments at 30 °C, 10 μl of protein sample was used and 20 μl for 40 °C. The protein sample was dispensed in a 384-well black flat transparent bottom plate (Nunc) and covered with 50 μl of mineral oil. The protein-containing wells were surrounded by buffer blanks dispensed in identical manner. Protein aggregation was measured for 7 days at 405 nm (using a Tecan Infinite M200 plate reader). Measurements were performed every minute for the first 5 h and every 30 min for the rest of the experiment. Solutions were homogenized by performing 3 s shaking before every measurement. TEV protease activity To assess the activity of the TEV protease WT and mutants, a substrate was designed: a fusion protein containing an N-terminal His6-tag and two SUMO subunits linked by a flexible (GGGS)2-ENLYFQ-(GGGS)2 linker (SUMO-TEV-SUMO). Thirty-five micrograms of substrate was mixed with 0.5 μg of TEV protease in a 25-μl reaction. The reaction was performed at RT, and 3 μl aliquots were removed at different time points. Substrate digestion was monitored by SDS–polyacrylamide gel electrophoresis. To determine activity after a heat challenge, the TEV protease sample was heated at 60 °C for 20 min before performing the activity assay as described. Accession codes: Coordinates and structure factors for NXR1-1 has been deposited in the RCSB protein data bank under accession code 4HVY . How to cite this article: Asial, I. et al . Engineering protein thermostability using a generic activity-independent biophysical screen inside the cell. Nat. Commun. 4:2901 doi: 10.1038/ncomms3901 (2013).